Co-option ofSox3as the male-determining factor on the Y chromosome in the fishOryzias dancena Sex chromosomes harbour a primary sex-determining signal that triggers sexual development of the organism. However, diverse sex chromosome systems have been evolved in vertebrates. Here we use positional cloning to identify the sex-determining locus of a medaka-related fish, Oryzias dancena , and find that the locus on the Y chromosome contains a cis -regulatory element that upregulates neighbouring Sox3 expression in developing gonad. Sex-reversed phenotypes in Sox3 Y transgenic fish, and Sox3 Y loss-of-function mutants all point to its critical role in sex determination. Furthermore, we demonstrate that Sox3 initiates testicular differentiation by upregulating expression of downstream Gsdf , which is highly conserved in fish sex differentiation pathways. Our results not only provide strong evidence for the independent recruitment of Sox3 to male determination in distantly related vertebrates, but also provide direct evidence that a novel sex determination pathway has evolved through co-option of a transcriptional regulator potentially interacted with a conserved downstream component. Most organisms have separate sexes, males and females, that differ not only in the primary reproductive organs but also in behavioural, morphological and physiological traits. In vertebrates, the phenotypic differences between the sexes are the result of differential expression of many genes during and after the development of testes or ovaries, whereas the sexual differentiation of the gonad is triggered by a primary sex-determining signal. However, these triggers are remarkably diverse, ranging from environmental to strict genetic cues, suggesting that new sex-determining signals have been generated repeatedly and frequently during vertebrate evolution [1] , [2] , [3] . Understanding the evolution of new sex determination mechanisms thus requires the identification of novel, primary sex-determining genes and the elucidation of differences in sexual differentiation molecular pathways. Relatively little is known, however, about primary genetic sex determination signals. Most experimental studies of primary genetic signals in vertebrates have been performed in well-developed model taxa having sex chromosomes. For example, the Y chromosome gene, Sry , is the master initiator for testicular development in mouse and human [4] , [5] , [6] , and is considered to have evolved from the X chromosomal Sox3 gene as an allelic variant on a proto-Y chromosome in the therian mammalian lineage [7] , [8] . However, Sry - or Sox3 -dependent sex determination has not been found in other vertebrates. Sex chromosome turnover is widespread in non-mammalian vertebrates, especially in fish [9] , [10] , suggesting that many different genes can act as the sex-determining signal. Several different sex-determining genes or candidates have been identified on the sex chromosomes of chicken [11] , frog [12] and fish [13] , [14] , [15] , [16] , [17] , [18] , but only rarely have they been formally demonstrated or their downstream pathways analysed. It is uncertain whether these genes are the major contributors to sex chromosome turnover, and it is unclear how these novel signals are integrated into the ancestral molecular pathway of sex determination. In contrast to the large diversity of primary sex-determining signals, it has been suggested that their downstream molecular components are typically more evolutionarily conserved [19] , [20] . The best example is Dmrt1 , which encodes a transcription factor that is broadly conserved in vertebrates and contains the DM domain (doublesex/mab-3 DNA-binding motif). Its male-specific upregulation has been observed in many taxa [21] , [22] , [23] , [24] , [25] , and it has been shown to be essential for testicular differentiation in mouse [26] , [27] , chicken [11] and medaka [28] . Many other genes involved in downstream pathways of mammalian sex differentiation have been found in the genomes of phylogenetically distant vertebrate taxa, although their functional conservation has not been determined. One promising model for understanding the evolution of sex-determining genes and pathways comprises the recently evolved sex determination mechanisms of medaka fishes in the genus Oryzias . Different sex chromosomes have been observed even in closely related fish species [29] , but most strikingly in the Oryzias fishes [30] , [31] , [32] , [33] , [34] . They show both XY and ZW systems, and their sex-determining loci are located on different chromosomes, suggesting that these mechanisms are regulated by different genes and have evolved rapidly. In a medaka-related fish, Oryzias dancena , sex is genetically determined by a single locus on the homomorphic XY chromosomes, although these sex chromosomes have no homology to those of any congeneric species examined so far [30] . Here we use the newly evolved Y chromosome of O. dancena to positionally clone and characterize its sex-determining locus, and to address how a novel sex-determining gene is generated and integrated into the developmental pathway of sexual differentiation. We identify the trigger responsible for sex determination, show that its novel expression in the developing gonad is induced by a cis -regulatory element at the sex-determining locus on the Y chromosome, and demonstrate that the novel sex determination pathway has evolved through the upregulation of a conserved downstream gene involved in testicular differentiation. Positional cloning of the sex-determining locus We have previously mapped the sex-determining locus of O. dancena within a genetic interval of 9.6 cM on its sex chromosomes, which are homologous to chromosome 10 of O. latipes [30] . To refine the position of the locus, we obtained additional siblings and genotyped novel markers within this interval to construct a high-resolution genetic map ( Fig. 1a ). We then constructed two bacterial artificial chromosome (BAC) libraries from YY and XX individuals, and performed chromosome walking on the Y and X chromosomes to develop BAC contigs anchored to the genetic map ( Fig. 1b ). These analyses defined a genetic interval of 0.1 cM between markers IMBY28J06R and Od38_01F , which was encompassed by three BAC clones on each of the Y and X chromosomes. These BAC clones were sequenced by the shotgun method, and we obtained draft sequences: a Y chromosomal region of 347,767 bp (mapped region: 309,526 bp) and an X chromosomal region of 323,094 bp (mapped region: 141,074 bp). To examine candidate genes, coding regions were identified using two different gene/exon prediction programs and by BLAST searches ( http://www.ncbi.nlm.nih.gov/BLAST/ ). 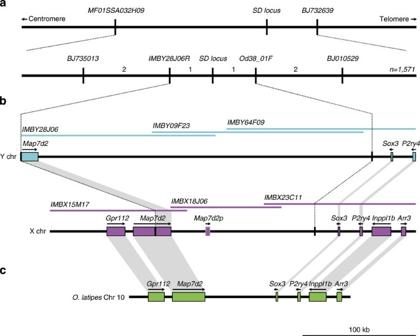Figure 1: Positional cloning of the sex-determining locus inO. dancena. (a) Genetic maps around the sex-determining (SD) locus. Numbers above the genetic map indicate the recombination events in 1,571 progeny. TheSDlocus was mapped within a genetic interval between two markers (IMBY28J06andF38_01F). (b,c) BAC contigs and physical maps of the Y and X chromosomes inO. dancena(b), and a physical map of the homologous sequence (6,885,000–7,080,000 bp) on chromosome 10 inO. latipes(c). Blue and purple lines indicate BAC clones; blue, purple and green boxes indicate genes; and arrows indicate the direction of transcription. Orthologous genes are connected by grey shading. Figure 1: Positional cloning of the sex-determining locus in O. dancena . ( a ) Genetic maps around the sex-determining ( SD ) locus. Numbers above the genetic map indicate the recombination events in 1,571 progeny. The SD locus was mapped within a genetic interval between two markers ( IMBY28J06 and F38_01F ). ( b , c ) BAC contigs and physical maps of the Y and X chromosomes in O. dancena ( b ), and a physical map of the homologous sequence (6,885,000–7,080,000 bp) on chromosome 10 in O. latipes ( c ). Blue and purple lines indicate BAC clones; blue, purple and green boxes indicate genes; and arrows indicate the direction of transcription. Orthologous genes are connected by grey shading. Full size image The sequence analysis revealed three genes ( Map7d2 , Sox3 and P2ry4 ) on the Y chromosome, and the same three genes plus additional three genes ( Gpr112 , Inppl1b and Arr3 ) and one pseudogene ( Map7d2p ) on the X chromosome ( Fig. 1b and Supplementary Table 1 ). All these genes were found on chromosome 10 of O. latipes with the same order and direction of transcription, confirming conserved synteny between the two species ( Fig. 1c and Supplementary Fig. 1 ). However, the genetically defined sex-determining region did not contain any coding sequences with similarity to known genes (except for the pseudogene on the X chromosome). Also in O. latipes , no predicted gene or cDNA was mapped within the region between Map7d2 and Sox3 ( Fig. 1c ). To investigate the genomic organization of the mapped region, we compared the Y and X chromosome sequences by dot-plot and VISTA plot. This analysis showed no similarity in the centre of the sequences, but detected a high degree of sequence conservation at both ends and numerous local duplications shared between the Y and X chromosomes ( Fig. 2a and Supplementary Fig. 2 ). The sequences with no homology suggest the presence of Y chromosome-specific insertions, while a large part of them consist of repetitive elements. A self-comparison of the Y chromosome sequence indicates that the mapped region consists largely of internal repetitive sequence blocks ( Fig. 2b ), which were rarely observed on the X chromosome ( Supplementary Fig. 3 ). Most of these blocks contain sequences that are not classified as known repetitive elements, and that showed no homology to the X chromosome sequence ( Fig. 2 ). Southern blot analysis of the sequences did not show any sex-specific hybridization pattern, suggesting that they were not particularly Y specific ( Supplementary Fig. 4 ). Furthermore, we identified known transposable elements within and between the internal repeat blocks using RepeatMasker, indicating that the Y-specific region was limited to very small intervals between such repetitive elements ( Fig. 2 , Supplementary Fig. 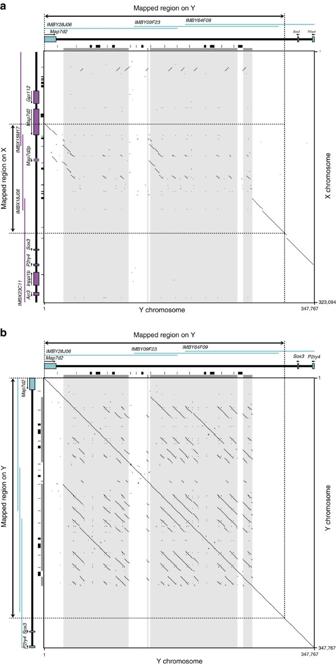Figure 2: Poor sequence homology of the sex-determining region between Y and X chromosomes. Dot-plots comparing the Y chromosome sequence to the X chromosome sequence (a), and the Y chromosome sequence to itself (b). The Y and X sequences are aligned at the left and right regions, but not in the middle of the Y chromosome region except for local duplications shared between the Y and X chromosomes (a). The single diagonal line in the Y–Y comparison shows that the sequence aligns over its entire length, and the smaller lines above and below the diagonal indicate multiple local duplications contained in this region of the Y chromosome (b). Blue and purple boxes indicate gene regions, and the arrows indicate the direction of transcription. Black boxes indicate known repeat regions detected by RepeatMasker, and grey boxes and shaded areas indicate the internal repeat regions on the Y chromosome. 1 and Supplementary Table 2 ). However, no Y-specific sequence was observed by Southern blot analyses using such interval sequences as probes ( Supplementary Fig. 4 ). These findings suggest that the mapped region consists of highly repetitive non-coding sequences, and that the differences between the Y and X chromosomes possibly contribute to sex determination in this species. Figure 2: Poor sequence homology of the sex-determining region between Y and X chromosomes. Dot-plots comparing the Y chromosome sequence to the X chromosome sequence ( a ), and the Y chromosome sequence to itself ( b ). The Y and X sequences are aligned at the left and right regions, but not in the middle of the Y chromosome region except for local duplications shared between the Y and X chromosomes ( a ). The single diagonal line in the Y–Y comparison shows that the sequence aligns over its entire length, and the smaller lines above and below the diagonal indicate multiple local duplications contained in this region of the Y chromosome ( b ). Blue and purple boxes indicate gene regions, and the arrows indicate the direction of transcription. Black boxes indicate known repeat regions detected by RepeatMasker, and grey boxes and shaded areas indicate the internal repeat regions on the Y chromosome. Full size image Functional analysis of the mapped region using transgenesis To test the mapped non-coding region for the ability to trigger sexual development, we generated transgenic O. dancena by introducing BAC clones, each of which partly covered the mapped region ( Fig. 3a ). We found that none of the BAC clones that contained only the mapped region induced any sex reversal phenotype. However, a Y chromosomal BAC clone ( IMBY64F09 ), which contained a part of the mapped region and the adjacent Sox3 and P2ry4 genes, induced sex-reversed XX males in two out of five independent transgenic lines. This BAC clone contained full coding sequences of Sox3 and P2ry4 , but did not include the P2ry4 upstream region. Furthermore, the Sox3 alleles on the Y and X chromosomes encoded the same amino-acid sequence ( Supplementary Fig. 5 ), suggesting that the BAC clone contained a cis -regulatory element of Sox3 that acts as a sex-determining signal, although this clone might not include the entire element. To investigate this further, we constructed a larger genomic clone ( BAC240 ) by joining two overlapping fosmid clones to a Y chromosomal BAC clone ( IMBY09F23 ). This clone also converted XX individuals into functional males in four out of four transgenic lines, reinforcing the presence of a male-determining function ( Fig. 3 ). In contrast, when the Sox3 coding region was replaced with an enhanced green fluorescent protein ( EGFP ) gene, no sex reversal was observed in either of two transgenic lines examined ( BAC240GFP ), supporting Sox3 -dependent sex determination. From these results, we concluded that a distant cis -regulatory element of Sox3 within the mapped region on the Y chromosome is required for male determination. 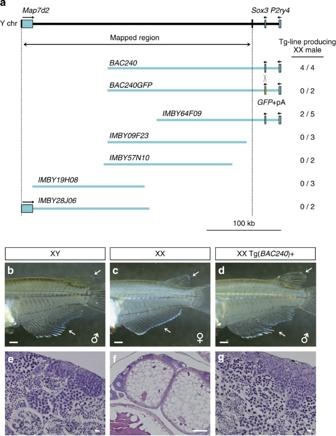Figure 3:Sox3-containing BAC clones caused XX sex reversal in transgenic fish. (a) Transgenic BAC constructs covering the sex-determining locus. Numbers indicate ratios of transgenic lines producing sex-reversed XX males to total lines. The large BAC,BAC240, was made by joining two overlapping fosmid clones toIMBY09F23, and the reporter constructBAC240GFPwas made by replacing the coding region ofSox3gene withGFP(green) followed by a BGH polyadenylation signal (pA). (b–d) Representative images of the external secondary sexual characteristics in control XY, XX and transgene (BAC240)-positive XX fish. The secondary sexual characteristics are manifested in the size and shape of dorsal and anal fins (arrows). Both dorsal and anal fins of males are larger than those of females. The transgene-positive XX fish developed as sex-reversed males (158/259 individuals in total). Scale bars, 1 mm. (e–g) Representative images of gonadal histology in control XY males (n=2), XX females (n=2) and the transgene-positive XX males (n=2). The sex-reversed XX males had normal testes. Scale bars, 10 μm (e,g); and 100 μm (f). Figure 3: Sox3 -containing BAC clones caused XX sex reversal in transgenic fish. ( a ) Transgenic BAC constructs covering the sex-determining locus. Numbers indicate ratios of transgenic lines producing sex-reversed XX males to total lines. The large BAC, BAC240 , was made by joining two overlapping fosmid clones to IMBY09F23 , and the reporter construct BAC240GFP was made by replacing the coding region of Sox3 gene with GFP (green) followed by a BGH polyadenylation signal (pA). ( b – d ) Representative images of the external secondary sexual characteristics in control XY, XX and transgene ( BAC240 )-positive XX fish. The secondary sexual characteristics are manifested in the size and shape of dorsal and anal fins (arrows). Both dorsal and anal fins of males are larger than those of females. The transgene-positive XX fish developed as sex-reversed males (158/259 individuals in total). Scale bars, 1 mm. ( e – g ) Representative images of gonadal histology in control XY males ( n =2), XX females ( n =2) and the transgene-positive XX males ( n =2). The sex-reversed XX males had normal testes. Scale bars, 10 μm ( e , g ); and 100 μm ( f ). Full size image Gonadal expression of Sox3 Sox3 encodes a transcription factor that contains a conserved high-mobility group domain, which is a characteristic feature of the SOX transcription factor family, and its expression is conserved in the central nervous system of vertebrate embryos [35] , [36] , [37] , [38] . Also, in O. dancena , Sox3 expression was observed in adult brain, eye and gill tissues, but not in mature ovary or testis ( Fig. 4a ). We then considered whether Sox3 expression in O. dancena was consistent with a role in gonadal sex determination. We examined its expression during early gonadal development by in situ hybridization, and found sexually dimorphic expression in the gonads ( Fig. 4b ). At 5 days post fertilization (d.p.f. ), Sox3 was expressed only in neural tubes and neuromasts in XX embryos, but additional signals were observed in somatic cells surrounding germ cells in XY gonads, supporting the notion that Sox3 has a critical role in testis determination. 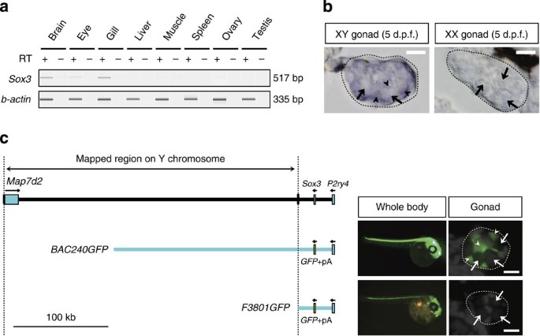Figure 4: Y chromosome-specificcis-regulatory element drivesSox3expression in developing gonads. (a) RT–PCR analysis ofSox3expression in adult tissues. A representative of two experiments is shown. (b)In situhybridization ofSox3mRNA in developing gonads of XY and XX embryos at 5 d.p.f. Images are representative of three gonads from each group.Sox3mRNA is localized in the somatic cells (arrowheads) surrounding germ cells (arrows) in the XY embryo but not in the XX embryo. (c) The reporter constructs, GFP expression in whole embryos and immunocytochemistry of GFP protein in gonad sections at 5 d.p.f.BAC240GFPdrove GFP expression in the somatic cells (arrowheads) surrounding germ cells (arrows), as well as in the neural tube and neuromasts (n=6), but the gonadal expression was not observed inOd38_01GFPtransgenic lines (n=4). Scale bars indicate 10 μm (b,c). Figure 4: Y chromosome-specific cis -regulatory element drives Sox3 expression in developing gonads. ( a ) RT–PCR analysis of Sox3 expression in adult tissues. A representative of two experiments is shown. ( b ) In situ hybridization of Sox3 mRNA in developing gonads of XY and XX embryos at 5 d.p.f. Images are representative of three gonads from each group. Sox3 mRNA is localized in the somatic cells (arrowheads) surrounding germ cells (arrows) in the XY embryo but not in the XX embryo. ( c ) The reporter constructs, GFP expression in whole embryos and immunocytochemistry of GFP protein in gonad sections at 5 d.p.f. BAC240GFP drove GFP expression in the somatic cells (arrowheads) surrounding germ cells (arrows), as well as in the neural tube and neuromasts ( n =6), but the gonadal expression was not observed in Od38_01GFP transgenic lines ( n =4). Scale bars indicate 10 μm ( b , c ). Full size image A cis -regulatory element induces gonadal Sox3 expression To examine the regulatory functions of the Y chromosome cis -regulatory element on gonadal Sox3 expression, we analysed reporter expression in transgenic lines bearing modified clones in which the Sox3 coding region was replaced with that of EGFP . The large BAC clone, BAC240GFP , modified from BAC240 , drove reporter expression in the developing gonads, as well as in the neural tube and neuromasts of XY individuals during early gonadal development in two independent transgenic lines ( Fig. 4c ). Gonadal reporter expression was observed at 5 d.p.f. but disappeared by the day of hatching (8 d.p.f. ), indicating its temporal expression in XY gonads ( Supplementary Fig. 6 ). In contrast, another clone that contained the genomic region surrounding Sox3 but that lacked the mapped region failed to drive gonadal reporter expression during development, although it could drive continuous expression in the neural tube and neuromasts in all three lines examined ( Fig. 4c ). Thus, the non-coding region downstream of Sox3 contains a tissue-specific cis -regulatory element that drives early gonadal expression only in XY individuals. Loss-of-function mutations of Sox3 Y cause XY sex reversal To confirm the role of Sox3 in sex determination, we knocked out the Sox3 gene using zinc-finger nuclease (ZFN) technology [39] because we could not target the cis -regulatory sequence. We designed ZFNs to target the N-terminal region of the Sox3 coding sequence ( Fig. 5a ), and injected mRNAs encoding the ZFNs into one-cell-stage embryos. We successfully obtained five independent mutant alleles having insertions or deletions at the target site: three X chromosome loss-of-function alleles ( X4ins , X13ins and X7del ) and two Y chromosome loss-of-function alleles ( Y4ins and Y16del ) ( Fig. 5b ). All five alleles caused frame shifts resulting in premature termination, predicted to yield proteins truncated in the high-mobility group domain ( Supplementary Fig. 7 ). We then examined the phenotypes of the mutant animals at 20 days post hatching (d.p.h.) and at the adult stage ( Fig. 5c–j and Supplementary Table 3 ). The gonads of heterozygous XX and XY fish with mutant alleles on the X chromosome revealed clear ovarian and testicular structures at 20 d.p.h., respectively, and they developed as fertile females or males according to their genotypic sex. In contrast, all heterozygous XY fish having the mutant alleles on the Y chromosome had ovary-type gonads at 20 d.p.h., and developed as fertile females. On the basis of this sex reversal phenotype, we concluded that Sox3 on the Y chromosome ( Sox3 Y ) is the male-determining gene in O. dancena . 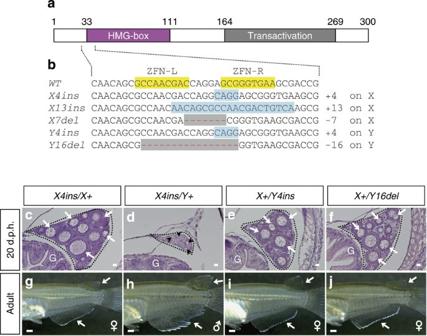Figure 5: Y chromosomal allele ofSox3is responsible for sex determination. (a) Representation of Sox3 protein inO. dancena. (b) Sequences of ZFN-induced mutant alleles. The wild-type sequence is shown at the top with ZFN half-sites highlighted in yellow. Insertions are indicated by blue-highlighted bold letters and deletions by grey-highlighted red dashes. (c–f) Histological sections of developing gonads inSox3heterozygous mutants at 20 d.p.h. Black arrowheads indicate gonial-type germ cells, and white arrowheads indicate various sizes of oocytes at the diplotene stage. XXSox3X4ins/+had an ovary with several oocytes (n=3) and XYSox3X4ins/+had a testis with spermatogonia (n=3), depending on their sex chromosome composition. In contrast, both XYSox3Y4ins/+(n=5) and XYSox3Y16del/+(n=6) had ovaries with oocytes. Scale bars, 10 μm. (g–j) The external secondary sexual characteristics of theSox3mutants at the adult stage. Both dorsal and anal fins of males are larger than those of females (arrows). XXSox3X4ins/+(n=45) and XYSox3X4ins/+(n=8) had female and male characters, respectively. But XYSox3Y4ins/+(n=6) and XYSox3Y16del/+(n=8) had female characters. Scale bars, 1 mm. Figure 5: Y chromosomal allele of Sox3 is responsible for sex determination. ( a ) Representation of Sox3 protein in O. dancena . ( b ) Sequences of ZFN-induced mutant alleles. The wild-type sequence is shown at the top with ZFN half-sites highlighted in yellow. Insertions are indicated by blue-highlighted bold letters and deletions by grey-highlighted red dashes. ( c – f ) Histological sections of developing gonads in Sox3 heterozygous mutants at 20 d.p.h. Black arrowheads indicate gonial-type germ cells, and white arrowheads indicate various sizes of oocytes at the diplotene stage. XX Sox3 X4ins/+ had an ovary with several oocytes ( n =3) and XY Sox3 X4ins/+ had a testis with spermatogonia ( n =3), depending on their sex chromosome composition. In contrast, both XY Sox3 Y4ins/+ ( n =5) and XY Sox3 Y16del/+ ( n =6) had ovaries with oocytes. Scale bars, 10 μm. ( g – j ) The external secondary sexual characteristics of the Sox3 mutants at the adult stage. Both dorsal and anal fins of males are larger than those of females (arrows). XX Sox3 X4ins/+ ( n =45) and XY Sox3 X4ins/+ ( n =8) had female and male characters, respectively. But XY Sox3 Y4ins/+ ( n =6) and XY Sox3 Y16del/+ ( n =8) had female characters. Scale bars, 1 mm. Full size image Conserved downstream pathway of sex determination in Oryzias In other Oryzias species, two male-determining genes have been isolated on different Y chromosomes. One is Dmy found in O. latipes [13] and the other is Gsdf in O. luzonensis [15] ( Supplementary Fig. 8 ). Dmy encodes a transcription factor containing a DM domain and Gsdf is a growth factor belonging to the transforming growth factor beta family. In O. latipes , Gsdf is expressed exclusively in XY somatic cells of developing gonads just after Dmy expression, indicating that Dmy acts upstream of Gsdf in the sex determination pathway [40] . In O. luzonensis , Dmy is absent, but the Y chromosome allele of Gsdf ( Gsdf Y ) is expressed earlier than the X chromosome allele, resulting in an XY-specific high level of Gsdf expression [15] . Both the Y and X alleles encode the same amino-acid sequence, suggesting that cis -regulatory mutations in the Gsdf Y promoter triggered its early gonadal expression, which led to establishment of its sex determination function without Dmy . We examined Gsdf expression in O. dancena , and found it to be expressed in an XY-specific manner during the early sex differentiation period ( Fig. 6a ). To elucidate the function of Sox3 in the sex determination pathway, we also analysed the expression of Gsdf in both the Sox3 Y gain-of-function transgenic fish and the Sox3 Y loss-of-function mutants, and found that Gsdf is expressed in gonadal somatic cells of the transgene-positive XX fish but not in the XY Sox3 Y4ins/+ mutants ( Fig. 6b ). Together, these data indicate that Sox3 acts upstream and is epistatic to Gsdf in the sex determination pathway. To further examine the role of Gsdf in testicular differentiation, we attempted to overexpress Gsdf in O. dancena developing gonads by introducing a genomic clone ( OluFY3-1 ) containing the Gsdf Y allele of O. luzonensis . This construct converted XX individuals into functional males in all five transgenic lines examined, suggesting a conserved role of Gsdf in testicular development ( Fig. 6c and Supplementary Table 4 ). Thus, these data suggest a model for an O. dancena sex determination pathway in which the early gonadal expression of Sox3 Y induces Gsdf expression directly or indirectly, allowing the bipotential gonads to develop as testes, resulting in the development of male individuals ( Supplementary Fig. 8 ). 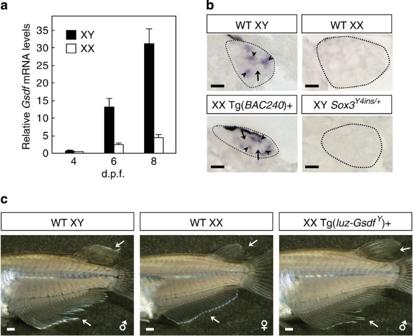Figure 6: Conserved role ofGsdfin male differentiation inOryziasspecies. (a) Quantitative real-time PCR ofGsdfexpression in three different stages (4–8 d.p.f.) ofO. dancenaembryos. Results are normalized toGapdhexpression and data are presented as mean±s.d. from three independent biological samples (one sample=pooled three embryos) for each of the stages. (b)In situhybridization ofGsdfmRNA in developing gonads of hatched fry at 8 d.p.f. Images are representative of four gonads from each group. In the wild type, strong signals forGsdfare seen in the somatic cells (arrowheads) surrounding the germ cells (arrows) in the XY fry but not in the XX fry. In contrast, its expression is induced in the gonads of XX Tg(BAC240)-positive sex reversal fish, and is totally abolished in those of XYSox3Y4ins/+loss-of-function mutants. (c) Representative images of the external secondary sexual characteristics in control XY, XX and transgene (luz-GsdfY)-positive XX fish at adult stage. Both dorsal and anal fins of males are larger than those of females (arrows). The transgene-positive XX fish developed as sex-reversed males (92/155 individuals in total; also seeSupplementary Table 4). Scale bars, 10 μm (b); 1 mm (c). Figure 6: Conserved role of Gsdf in male differentiation in Oryzias species. ( a ) Quantitative real-time PCR of Gsdf expression in three different stages (4–8 d.p.f.) of O. dancena embryos. Results are normalized to Gapdh expression and data are presented as mean±s.d. from three independent biological samples (one sample=pooled three embryos) for each of the stages. ( b ) In situ hybridization of Gsdf mRNA in developing gonads of hatched fry at 8 d.p.f. Images are representative of four gonads from each group. In the wild type, strong signals for Gsdf are seen in the somatic cells (arrowheads) surrounding the germ cells (arrows) in the XY fry but not in the XX fry. In contrast, its expression is induced in the gonads of XX Tg( BAC240 )-positive sex reversal fish, and is totally abolished in those of XY Sox3 Y4ins/+ loss-of-function mutants. ( c ) Representative images of the external secondary sexual characteristics in control XY, XX and transgene ( luz-Gsdf Y )-positive XX fish at adult stage. Both dorsal and anal fins of males are larger than those of females (arrows). The transgene-positive XX fish developed as sex-reversed males (92/155 individuals in total; also see Supplementary Table 4 ). Scale bars, 10 μm ( b ); 1 mm ( c ). Full size image We have shown that the Y chromosome allele of Sox3 is both required and sufficient for male determination in O. dancena , and its essential expression in the developing gonad is driven by a distant cis -regulatory element at the sex-determining locus on the Y chromosome. This suggests that the new Y chromosome of O. dancena arose by co-option of the Sox3 gene. A similar evolutionary process is thought to have occurred in mammals, in which the male-determining gene, Sry is considered to have evolved from Sox3 through a regulatory mutation in the proto-Y chromosome allele [7] . This hypothesis has been strongly supported by recent studies of Sox3 transgenic mice and human sex reversal cases. Ectopic expression of Sox3 in the urogenital ridge of transgenic mice induces complete XX male sex reversal [8] , and rearrangements in the Sox3 regulatory region are associated with XX male sex reversal in human [8] , [41] , suggesting that Sry and Sox3 are functionally interchangeable in sex determination. Thus, although loss of Sox3 function does not affect sex determination [42] , certain gain-of-function mutations in Sox3 may result in XX male sex reversal in mouse and human by mimicking the function of Sry , supporting the notion that Sry evolved from Sox3 (ref. 7 ). These findings suggest that the same Sox3 gene has been independently recruited for generating a novel Y chromosome in distantly related vertebrates, a medaka-related species and therian mammals. The repeated appearance of homologous chromosomes or genomic regions involved in sex determination has been observed in other vertebrates, suggesting that the same genes may have independently acquired the function of sex determination [2] . The repeated association of Sox3 with the generation of new sex chromosomes seems to have also occurred in other vertebrate species, such as the wrinkled frog [43] . Similarly, Dmrt1 is a strong candidate for the sex-determining gene in chicken [11] , and its paralogues, Dmy [13] and Dm-W 12 , have evolved as male- and female-determining genes in medaka and Xenopus laevis , respectively. Such Sox3 - and Dmrt1 -related genes may be suitable for generating new sex-determining genes [2] , although they are not the only genes that can act as the trigger. Recent reports show that a few regulatory or coding mutations in other pre-existing and duplicated genes can generate new sex-determining genes in fishes [14] , [15] , [16] . For example, a few Y chromosome-specific nucleotide changes in the cis -regulatory region of Gsdf Y contribute to its male-specific high level of expression leading to testicular development in a medaka-related fish, O. luzonensis [15] . Furthermore, a missense single-nucleotide polymorphism in Amhr2 is the only difference associated with phenotypic sex in fugu [16] . Thus, it is very likely that co-option of the same genes, as we have demonstrated here in O. dancena , has contributed to the remarkable variety of sex determination signals and sex chromosomes in vertebrates. We have not yet identified the Y chromosome-specific cis -regulatory sequence at the sex-determining locus that dominantly affects distant Sox3 expression. However, our transgenic experiments have clearly demonstrated that the genetically mapped region contains a distal regulatory element(s), which may be an enhancer acting as a transcription factor binding site or a recently described non-coding RNA displaying enhancer-like activity via a cis -mediated mechanism [44] , [45] , [46] . The mapped region contains a large number of repetitive sequences, such as the tandemly arrayed large internal repeats and known transposable elements. Sequence comparison of this region between the Y and X chromosomes suggested Y chromosome-specific repetitive and unique sequences, but neither was found to be Y specific by Southern blot experiments, thereby suggesting that this region consists largely of the interspersed repetitive sequences dispersed throughout the O. dancena genome. It has been proposed that insertions of such transposable elements are potential sources of new cis -regulatory elements [47] , [48] and long non-coding RNAs [49] , [50] . Transposable elements are abundant in vertebrate genomes, and some of them have been shown to function as cis -regulatory elements of specific genes [51] , [52] , [53] . It is also possible that in O. dancena , the Y chromosome-specific insertion or accumulation of repetitive elements has served as the distant cis -regulatory sequence driving Sox3 expression. We have also demonstrated that Sox3 evolved as the sex-determining gene in O. dancena by activating a downstream Gsdf gene, which is considered to be a key component of the male differentiation pathway in fish. Gsdf is a recently described member of the transforming growth factor beta family detected only in teleosts [54] . In Oryzias , Gsdf ( Gsdf Y ) functions as the male-determining gene in O. luzonensis [15] , and another male-determining gene, Dmy , activates Gsdf expression during early gonadal development in O. latipes [40] . In addition, our transgenic experiments showed that Gsdf Y of O. luzonensis induced sex-reversed XX males in O. dancena , as well as in O. latipes [15] . Also in another fish species, sablefish, Gsdf is located on its sex chromosomes, and shows male-specific high expression levels [18] . Furthermore, higher levels of Gsdf expression in testis have been observed in other distantly related fishes, including zebrafish [55] , [56] , three-spot wrasse [57] and coelacanth [58] , suggesting that this gene arose before the divergence of fish and tetrapod lineages, and might be a key ancestral factor for testis differentiation [58] . Therefore, such conserved downstream components and their potential transcriptional regulators might have been major contributors to the generation of a novel sex determination pathway. Fish and sexing Wild stocks of O. dancena originally collected at Chidambaram, India (Strain ID: RS274) and Phuket, Thailand (ID: RS275) were supplied by the National BioResource Project (Medaka) ( http://www.shigen.nig.ac.jp/medaka/ ). The fish were maintained in aquaria under an artificial 14 h light:10 h dark photoperiod at 27±2 °C. All animal experiments complied with the guideline of National Institute for Basic Biology, and were approved by the Institutional Animal Care and Use Committee of National Institute of Natural Science (the approval IDs: 09A184, 10A212, 12A087 and 13A156). Phenotypic sex was judged on the basis of secondary sex characteristics, namely, the shapes of the dorsal and anal fins at 2 months after hatching. Genotypic sex (XX or XY) was determined by PCR genotyping of two sex-linked markers ( BJ010529 and BJ735013 ) using a high-resolution melting assay. Primer sequences are listed in Supplementary Table 5 . Positional cloning of the sex-determining locus Linkage analysis was performed using backcross progeny between Chidambaram and Phuket stocks of O. dancena as described previously [30] . To identify recombinants around the sex-determining locus, we isolated genomic DNA from 1,571 fish of the backcross population and genotyped two novel markers ( BJ010529 and BJ735013 ) according to the draft genome sequence of O. latipes . To further determine the location of the sex-determining locus, we generated BAC-end sequence-derived markers according to the physical map and determined genotypes of the recombinants with these markers. The primer sequences used in this study are listed in Supplementary Table 5 . Construction of BAC library and chromosome walking To generate physical maps around the sex-determining locus, BAC genomic DNA libraries, IMBX and IMBY, were constructed from XX and YY embryos of O. dancena , respectively. The genomic DNA was partially digested with Sac I, and fragments in the size range of 150–225 kb were isolated. The size-selected DNA fragments were ligated into pKS145 and used to transform DH10B. For each library, a total of 36,864 clones were picked and arrayed into 96 × 384-well microtiter plates. Using a systematic PCR-based procedure, these libraries were screened with the sex-determining locus flanking markers, BJ010529 and BJ73501 3. Sequences from the ends of individual clones were determined by cycle sequencing using M13 primers. Primers designed to BAC-end sequences were used in genetic mapping and subsequent screening of the BAC libraries. Primer sequences are listed in Supplementary Table 5 . To fill gaps between BAC clones, we also used a fosmid library [30] constructed from an O. dancena XY individual. Sequence analysis Three Y chromosome BAC clones ( IMBY09F23 , IMBY28J06 and IMBY64F09 ) and three X chromosome clones ( IMBX15M17 , IMBX18J06 and IMBX23C11 ) were sequenced using a shotgun sequencing procedure and assembled using the Parallel Contig Assembly Program ( http://seq.cs.iastate.edu/ ). However, two Y chromosome clones ( IMBY09F23 and IMBY28J06 ) were poorly assembled owing to numerous internal repeat sequences. To resolve the assembly of the two clones, we obtained PacBio long reads and assembled using the Hierarchical Genome Assembly Process. After assembly, gene annotation was performed using gene prediction software (GENSCAN; http://genes.mit.edu/GENSCAN.html and FGENESH; http://www.softberry.com/berry.phtml ). Homology to known genes was determined using BLAST against the non-redundant database in GenBank ( http://www.ncbi.nlm.nih.gov/blast/Blast.cgi ). The positions of exons of known genes were identified based on full-length cDNA sequences in the National BioResource Project genome database of O. latipes ( http://www.shigen.nig.ac.jp/medaka/ ) or the predicted coding sequences in the NCBI database. To identify known repetitive elements, the sequences were analysed with RepeatMasker 4.0.3 ( http://www.repeatmasker.org/ ) (RM database version 20130422). A global pairwise alignment of the Y and X chromosome sequences was performed using mVISTA ( http://genome.lbl.gov/vista/index.shtml ) with 70% stringency, 100 bp window size and fugu repetitive element masking. Dot-plot analysis was performed with the software, Dotter ( http://sonnhammer.sbc.su.se/Dotter.html ). Transgenic constructs and microinjection BAC and fosmid clones were modified by homologous recombination in Escherichia coli as described [59] . To facilitate the pre-selection of transgenic embryos, the reporter gene cassette (crystallin-gM2-hrGFP) was amplified via PCR from a vas-GFPnuc-cryGFP plasmid and inserted into the BAC-vector backbone. Primers used for BAC modification are listed in Supplementary Table 5 . To construct the large BAC clone ( BAC240 ), we joined a BAC clone ( IMBY09F23 ) to two overlapping fosmid clones ( Od38_01 and Od39_01 ) by iterative recombination. To generate BAC240GFP and F3801GFP clones, the Sox3 gene region was replaced with an EGFP+polyA cassette PCR amplified from the hsGBA-NKm plasmid [60] , [61] . For efficient BAC and fosmid transgenesis using the medaka Tol2 transposon, we inserted the iTol2 cassette into the vector backbone of all clones [62] , [63] . Each modified clone was purified using a Qiagen Large-Construct kit (Qiagen), and Tol2 transposon mRNA was synthesized in vitro using an SP6 mMessage mMachine kit (Ambion). The BAC DNA and the Tol2 mRNA were co-injected into one-cell-stage embryos of O. dancena , and independent stable lines were obtained for each clone. In situ hybridization and immunohistochemistry Embryos were fixed in 4% paraformaldehyde in PBS at 4 °C overnight. For in situ hybridization, digoxigenin (DIG)-labelled RNA probes were generated by in vitro transcription with a DIG RNA labelling kit (Roche) from a Sox3 or a Gsdf plasmid. Sections were deparaffinized, hydrated, treated with proteinase K (10 mg ml −1 ) at 37 °C for 5 min, and hybridized with the DIG-labelled antisense RNA probes at 60 °C for 18–24 h. Hybridization signals were detected using an alkaline phosphatase-conjugated anti-DIG antibody (Roche, cat. no. 11093274910, 1/1,000 diluted) with nitroblue tetrazolium chloride (NBT)/5-bromo-4-chloro-3-indolyl-phosphate, 4-toluidine salt (BCIP) (Roche) as the chromogen. For immunohistochemistry, we used rabbit anti-GFP (Invitrogen, cat. no. A11122, 1:500 diluted) and anti-rabbit/Alexa Fluor 488-conjugated antibodies (Invitrogen, cat. no. A21206, 1/1,000 diluted) as primary and secondary antibodies, respectively. Histological observation of gonads Tissue samples were fixed in Bouin’s solution overnight, dehydrated in a series of ethanol solutions and embedded in paraffin. Cross-sections of the body portion containing a whole gonad were cut serially at 5 mm thickness and stained with hematoxylin and eosin. Sections of the gonad were observed carefully under an Olympus BX50 light microscope and were captured with a DP71 digital camera. Reverse transcription PCR and quantitative reverse transcription PCR Total RNA was extracted from adult tissues or embryos with RNeasy (Qiagen). Contaminating DNA was removed by DNaseI treatment (Qiagen). First strand cDNA was synthesized from 150 ng of total RNA with Omni-script reverse transcriptase (Qiagen). Reverse transcription (RT) PCR conditions were as follows: 30 s at 96 °C, 30 s at the annealing temperature and 60 s at 72 °C. The number of PCR cycles for Sox3 and b-actin were adjusted to be 30 and 24 cycles, and the annealing temperature at 60 °C and 55 °C, respectively. RT–PCR products were analysed using the MultiNA microchip electrophoresis system (Shimadzu). The MultiNA gel image is presented in Supplementary Fig. 9 . Quantitative RT-PCR was performed in an optical 96-well plate with an ABI 7500 Real-Time PCR System (Applied Biosystems) using a KAPA SYBR Fast qPCR Kit (Kapa Biosystems) according to the manufacturer’s instructions. Cycling conditions were as follows: 95 °C for 30 s; 40 cycles of 95 °C for 5 s and 60 °C for 34 s. PCR amplification specificity was verified against a dissociation curve (60–95 °C). Expression levels of Gsdf were normalized to the values for Gapdh . Three independent experiments were performed in all cases. Data were analysed using 7500 software (Applied Biosystems). Primer sequences used are listed in Supplementary Table 5 . ZFN constructs and mutation screening ZFNs were engineered using context-dependent assembly [39] . ZFN target sites in the endogenous Sox3 sequence of O. dancena were identified using the publicly available Web-based programme, ZiFiT Targeter ( http://zifit.partners.org/ZiFiT/ ). Left and right zinc-finger arrays were assembled by PCR and cloned into pMLM290 or pMLM292 expression vectors that encode Fok I nuclease. In vitro transcription of ZFN mRNA for injection was conducted by linearizing the expression plasmids with Pme I, and transcribing the linearized DNA using a T7 mMessage mMachine kit (Ambion). One-cell-stage embryos were microinjected with 25 ng μl −1 of ZFN mRNA, and injected fish were mated with normal fish to obtain progeny. Genomic DNA was isolated from the F 1 progeny, and genotyped by a high-resolution melting assay and/or sequencing of the PCR-amplified target region. Primer sequences are listed in Supplementary Table 5 . Accession codes: cDNA sequences of Sox3 and genomic DNA sequences of the sex-determining region on X and Y chromosomes of O. dancena have been deposited at DDBJ/GenBank under accession numbers AB775142 , AB775143 , AB909496 and AB909497 . How to cite this article: Takehana, Y. et al. Co-option of Sox3 as the male-determining factor on the Y chromosome in the fish Oryzias dancena . Nat. Commun. 5:4157 doi: 10.1038/ncomms5157 (2014).